Hypothalamic proteoglycan syndecan-3 is a novel cocaine addiction resilience factor Proteoglycans like syndecan-3 have complex signaling roles in addition to their function as structural components of the extracellular matrix. Here, we show that syndecan-3 in the lateral hypothalamus has an unexpected new role in limiting compulsive cocaine intake. In particular, we observe that syndecan-3 null mice self-administer greater amounts of cocaine than wild-type mice. This effect can be rescued by re-expression of syndecan-3 in the lateral hypothalamus with an adeno-associated viral vector. Adeno-associated viral vector delivery of syndecan-3 to the lateral hypothalamus also reduces motivation for cocaine in normal mice. Syndecan-3 limits cocaine intake by modulating the effects of glial-cell-line-derived neurotrophic factor, which uses syndecan-3 as an alternative receptor. Our findings indicate syndecan-3-dependent signaling as a novel therapeutic target for the treatment of cocaine addiction. Addiction is a chronic relapsing disorder characterized by compulsive drug seeking, loss of control over drug intake and dysregulation of reward and emotional systems. Multiple factors have been identified that convey vulnerability to cocaine addiction including dysregulation of the mesolimbic dopamine system and activation of brain stress systems [1] , [2] , [3] . However, few, if any, studies have identified addiction-resistant factors. Syndecans are cell-associated heparan sulfate proteoglycans characterized by cysteine-free extracellular domains that extend from the cell surface, allowing them to act as either co-receptors or alternative receptors for several peptides such as glial cell line-derived neurotrophic factor (GDNF), fibroblast growth factors, pleiotrophin, midkine, vascular endothelial growth factors, and transforming growth factor-β, as well as extracellular matrix proteins like fibronectin and laminin [4] , [5] , [6] , [7] . Four mammalian syndecans have been identified, of which syndecan-3, also known as N -Syndecan, is enriched in the brain [4] . The hypothalamus has a crucial role in reward processing and addictive behaviors as part of the key circuitry of the mesocorticolimbic dopamine system and the extended amygdala that mediate the reinforcing actions of cocaine and other drugs of abuse. In fact, the lateral hypothalamus (LH) is heavily interconnected with extended amygdala and basal forebrain regions involved in drug reward and dependence [8] , and gene expression profiling showed evidence of a substantial remodeling of LH circuitry associated with the transition from controlled to compulsive cocaine self-administration [9] . Using syndecan-3 knockout (KO) mice and adeno-associated (AAV) viral vector to re-express syndecan-3, we show that syndecan-3 in the LH has a role in limiting compulsive cocaine intake by modulating GDNF actions. Our findings indicate syndecan-3-dependent signaling as a novel therapeutic target for the treatment of cocaine addiction. Cocaine induces syndecan-3 in the lateral hypothalamus Microarray analyses revealed that a history of cocaine self-administration increased syndecan-3 mRNA in the rat LH but not in the nucleus accumbens (NAc) ( Fig. 1a and Supplementary Fig. S1 ). Using the GSEA algorithm for pathway analysis, we observed that genes involved in syndecan-3-dependent signaling were significantly differentially expressed in the rat LH by cocaine, indicating that cocaine induces changes in the regulation of syndecan-3-dependent signaling (NES=1.9, P -value<0.001; Fig. 1b and Supplementary Table S1 ). Similarly, cocaine significantly increased syndecan-3 mRNA ( Fig. 1c ) and protein ( Supplementary Fig. S2 ) in the mouse LH and in the LH of cocaine-self-administering macaques ( Fig. 1d ). 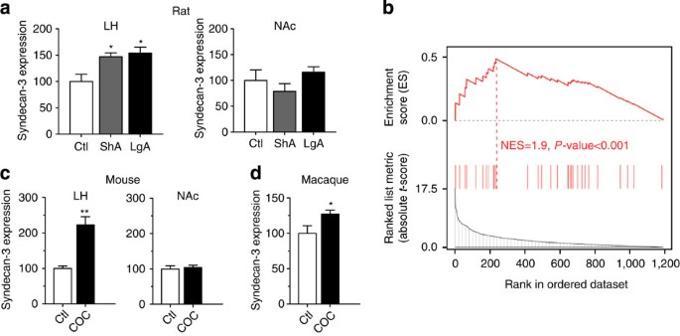Figure 1: LH syndecan-3 is induced by cocaine. (a) Syndecan-3 is induced by cocaine intake in the LH, but not in the NAc of cocaine-self-administering rats as measured by quantitative real-time PCR (qRT-PCR) with the standard curve method normalizing to β-actin (n=4–5). Units on theyaxis represent the ratios of syndecan mRNA levels to that of β-actin in each region (*P<0.05, by one-way ANOVA with Tukey’spost-hoctest). (b) GSEA indicates that genes related to syndecan-3-dependent signaling are enriched in differentially expressed genes in the LH of cocaine-self-administering rats compared with control rats (normalized enrichment score, NES=1.9;P<0.001). The dotted line, also called leading edge, indicates the point at which the running enrichment score reaches its maximum score. (c) Cocaine increases the expression of syndecan-3 mRNA in the LH but not in the NAc of mice after six daily IP administrations of 18 mg kg−1of cocaine; control mice received isovolemic injections of saline vehicle (n=5; **P<0.01 byt-test). (d) Syndecan-3 mRNA is increased in the LH in cocaine-self-administering macaques (n=4; *P<0.05 byt-test). Data are presented as mean±s.e.m. Figure 1: LH syndecan-3 is induced by cocaine. ( a ) Syndecan-3 is induced by cocaine intake in the LH, but not in the NAc of cocaine-self-administering rats as measured by quantitative real-time PCR (qRT-PCR) with the standard curve method normalizing to β-actin ( n =4–5). Units on the y axis represent the ratios of syndecan mRNA levels to that of β-actin in each region (* P <0.05, by one-way ANOVA with Tukey’s post-hoc test). ( b ) GSEA indicates that genes related to syndecan-3-dependent signaling are enriched in differentially expressed genes in the LH of cocaine-self-administering rats compared with control rats (normalized enrichment score, NES=1.9; P <0.001). The dotted line, also called leading edge, indicates the point at which the running enrichment score reaches its maximum score. ( c ) Cocaine increases the expression of syndecan-3 mRNA in the LH but not in the NAc of mice after six daily IP administrations of 18 mg kg −1 of cocaine; control mice received isovolemic injections of saline vehicle ( n =5; ** P <0.01 by t -test). ( d ) Syndecan-3 mRNA is increased in the LH in cocaine-self-administering macaques ( n =4; * P <0.05 by t -test). Data are presented as mean±s.e.m. Full size image Syndecan-3 regulates cocaine intake To test the hypothesis that syndecan-3 may regulate cocaine intake, we first investigated cocaine self-administration in mice lacking syndecan-3. Syndecan-3 KO and wild-type mice were trained to self-administer cocaine in daily 1 h sessions under a fixed ratio 1 schedule (FR1), whereby each lever press resulted in an injection of 0.6 mg per kg of cocaine. As shown in Fig. 2a , syndecan-3 KO mice acquired intravenous cocaine self-administration at a similar rate as wild-type mice, but self-administered greater amounts of cocaine after acquisition of self-administration on testing days 8–12. After 12 1-h daily sessions of cocaine self-administration, syndecan-3 KO and wild-type mice were compared in cocaine unit dose-response curves under an FR5 schedule, which increases the amount of work needed to obtain a reward. Results showed that the cocaine dose-response curve was shifted upward in syndecan-3 null mice when compared with wild-type mice ( Fig. 2b ), and that syndecan-3 null mice consumed greater amounts of cocaine as the dose increased from 0.15 to 1.2 mg per kg per infusion ( Fig. 2c ). An upward shift in the inverted U-shaped dose-response curve is associated with greater vulnerability to abuse cocaine in animal models [10] . This effect was specific as syndecan-3 null and wild-type mice did not differ in preference for a natural reward like sucrose over a broad range of concentrations ( Fig. 3 ). In agreement with this finding, syndecan-3 null mice consumed less of a high-fat food than wild-type mice [11] and showed enhanced sensitivity to anorexigenic agents [12] . Syndecan-3 null and wild-type mice also did not differ in the locomotor and cardiovascular effects of cocaine, as measured by EKG, suggesting that differences in rates of cocaine self-administration could not be explained by differences in the stimulatory and cardiovascular effects of the drug ( Supplementary Figs. S3 and S4 ). Thus, syndecan-3 null mice self-administer greater amounts of cocaine and show increased cocaine seeking. 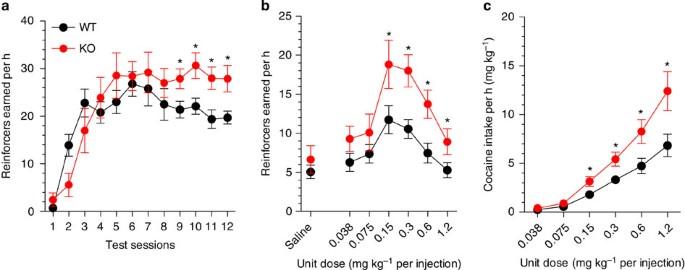Figure 2: Syndecan-3 deficiency increases cocaine intake. (a) Acquisition of intravenous cocaine self-administration (FR1) in wild-type (WT) and syndecan-3 KO mice. Following acquisition, syndecan-3 KO mice showed a higher level of cocaine intake at the training dose (FR1). Repeated measures (RM) two-way ANOVA: Test sessionF(11,187)=19.15,P<0.0001; GenotypeF(1,187)=2.343,P=0.144; InteractionF(1,187)=2.233,P=0.014. (b) The dose-response curve (FR5) of syndecan-3 KO mice was upward-shifted compared with WT mice. DoseF(6,120)=29.78,P<0.0001; GenotypeF(1,120)=4.621,P=0.044; InteractionF(6,120)=3.137,P=0.007. (c) Dose-intake curve (same mice as in middle panel). Syndecan-3 KO mice self-administered greater amounts of cocaine. DoseF(5,85)=59.26,P<0.0001; GenotypeF(1,85)=7.793,P=0.013; InteractionF(5,85)=4.958,P<0.001. Data are presented as mean±s.e.m. *P<0.05 compared with wild-type mice (LSD post-hoc test;n=9–10). Figure 2: Syndecan-3 deficiency increases cocaine intake. ( a ) Acquisition of intravenous cocaine self-administration (FR1) in wild-type (WT) and syndecan-3 KO mice. Following acquisition, syndecan-3 KO mice showed a higher level of cocaine intake at the training dose (FR1). Repeated measures (RM) two-way ANOVA: Test session F (11,187) =19.15, P <0.0001; Genotype F (1,187) =2.343, P= 0.144; Interaction F (1,187) =2.233, P =0.014. ( b ) The dose-response curve (FR5) of syndecan-3 KO mice was upward-shifted compared with WT mice. Dose F (6,120) =29.78, P <0.0001; Genotype F (1,120) =4.621, P =0.044; Interaction F (6,120) =3.137, P =0.007. ( c ) Dose-intake curve (same mice as in middle panel). Syndecan-3 KO mice self-administered greater amounts of cocaine. Dose F (5,85) =59.26, P <0.0001; Genotype F (1,85) =7.793, P =0.013; Interaction F (5,85) =4.958, P <0.001. Data are presented as mean±s.e.m. * P <0.05 compared with wild-type mice (LSD post-hoc test; n =9–10). 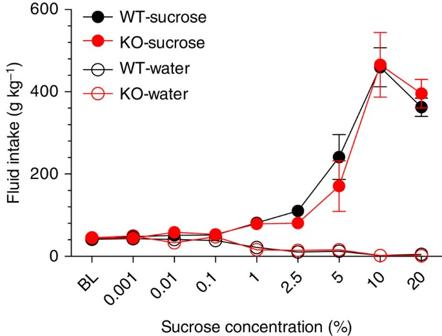Figure 3: Syndecan-3 deficiency does not affect sucrose intake. Sucrose consumption was not different in syndecan-3 KO and wild-type (WT) mice over a broad range of sucrose concentrations as assessed by a two- bottle choice procedure. Both syndecan-3 KO and wild-type mice showed dose-related increase in sucrose intake (n=12 for each group). Data are presented as mean±s.e.m. Full size image Figure 3: Syndecan-3 deficiency does not affect sucrose intake. Sucrose consumption was not different in syndecan-3 KO and wild-type (WT) mice over a broad range of sucrose concentrations as assessed by a two- bottle choice procedure. Both syndecan-3 KO and wild-type mice showed dose-related increase in sucrose intake ( n =12 for each group). Data are presented as mean±s.e.m. Full size image To confirm the hypothesis that the deficiency of syndecan-3 in the LH results in enhanced responding for cocaine in syndecan-3 null mice, we used an AAV vector to re-express syndecan-3 in the LH of these mice ( Fig. 4a ). As syndecan-3-dependent signaling is terminated by ectodomain shedding [13] , we used a shedding-resistant allele of syndecan-3. We observed that expression of this modified syndecan-3 in the LH of syndecan-3 KO mice downward-shifted the dose-response curves and reduced cocaine intake when compared with syndecan-3 null mice injected in the LH with control GFP-expressing AAV ( Fig. 4b ). This indicates that LH syndecan-3 is key in the increased reinforcing properties of cocaine that we observed in syndecan-3 null mice and that the phenotype is unlikely to result from a developmental defect. We then investigated the effect of LH overexpression of syndecan-3 on cocaine self-administration by wild-type mice. To this end, AAV expressing either the shedding-resistant syndecan-3 or GFP were injected in the LH of wild-type mice, and then tested in cocaine self-administration with a progressive ratio (PR) schedule of reinforcement, whereby the cost for each injection increases progressively. Cocaine injections earned under PR conditions are considered to be an indicator of the amount of effort an animal is willing to expend to obtain a cocaine reward, and increased responding on a PR schedule is considered a measure of compulsivity. As shown in Fig. 4c , injection of syndecan-3-expressing AAV dramatically downward-shifted the dose-response curves of wild-type mice under the PR schedule of reinforcement, indicating that LH syndecan-3 regulates motivation for cocaine also in normal mice. 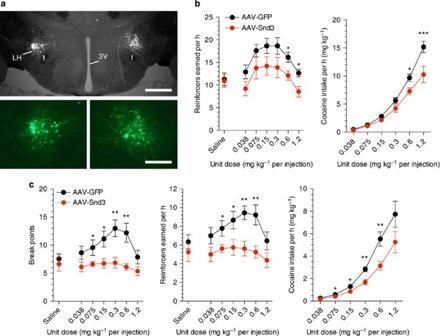Figure 4: Rescue of syndecan-3 expression in the LH reduces cocaine intake in syndecan-3 KO mice. (a) Immunochemical staining for GFP of a mouse infused with AAV in the LH; Scale bar correspond to 400 μm in the top panel and 200 μm in the bottom ones; (b) Left panel: Intra-LH infusions of AAV-Snd3 downward-shifted the dose-response curve in syndecan-3 KO mice (FR5). DoseF(6,102)=10.55,P<0.0001; AAV-Snd3F(1,102)=4.596,P=0.047. Right panel: The dose-intake curve was shifted downward in AAV-Snd3-infused syndecan-3 KO mice (same mice as in left panel). DoseF(5,85)=148.4,P<0.0001; AAV-Snd3F(1,85)=9.135,P=0.008; Interaction F(5,85)=5.443,P<0.001.n=9–10. (c) Left panel: Wild-type mice receiving intra-LH AAV-Snd3 reached lower breakpoints than AAV-GFP mice under a PR schedule. DoseF(6,90)=3.55,P=0.003; AAV-Snd3F(1,90)=10.51,P=0.006; Interaction F(6,90)=2.311,P=0.04. Middle panel: the dose-response curve of wild-type mice was shifted downward by AAV-Snd3. DoseF(6,90)=3.415,P=0.004; AAV-Snd3F(1,90)=9.075,P=0.009. Right: dose-intake curve was reduced by AAV-Snd3 in wild-type mice. DoseF(5,75)=60.09,P<0.0001; AAV-Snd3F(5,75)=7.638,P=0.015; InteractionF(5,75)=2.915,P=0.019.n=8–9. Data are presented as mean±s.e.m. *P<0.05 and **P<0.01, AAV-GFP-infused versus AAV-Snd3-infused mice (LSDpost-hoctest). Figure 4: Rescue of syndecan-3 expression in the LH reduces cocaine intake in syndecan-3 KO mice. ( a ) Immunochemical staining for GFP of a mouse infused with AAV in the LH; Scale bar correspond to 400 μm in the top panel and 200 μm in the bottom ones; ( b ) Left panel: Intra-LH infusions of AAV-Snd3 downward-shifted the dose-response curve in syndecan-3 KO mice (FR5). Dose F (6,102) =10.55, P <0.0001; AAV-Snd3 F (1,102) =4.596, P =0.047. Right panel: The dose-intake curve was shifted downward in AAV-Snd3-infused syndecan-3 KO mice (same mice as in left panel). Dose F (5,85) =148.4, P <0.0001; AAV-Snd3 F (1,85) =9.135, P =0.008; Interaction F (5,85) =5.443, P <0.001. n =9–10. ( c ) Left panel: Wild-type mice receiving intra-LH AAV-Snd3 reached lower breakpoints than AAV-GFP mice under a PR schedule. Dose F (6,90) =3.55, P =0.003; AAV-Snd3 F (1,90) =10.51, P =0.006; Interaction F (6,90) =2.311, P =0.04. Middle panel: the dose-response curve of wild-type mice was shifted downward by AAV-Snd3. Dose F (6,90) =3.415, P =0.004; AAV-Snd3 F (1,90) =9.075, P =0.009. Right: dose-intake curve was reduced by AAV-Snd3 in wild-type mice. Dose F (5,75) =60.09, P <0.0001; AAV-Snd3 F (5,75) =7.638, P =0.015; Interaction F (5,75) =2.915, P =0.019. n =8–9. Data are presented as mean±s.e.m. * P <0.05 and ** P <0.01, AAV-GFP-infused versus AAV-Snd3-infused mice (LSD post-hoc test). Full size image Syndecan-3 modulates the effects of GDNF on cocaine intake One of the key roles of syndecans is to bind growth factors through their glycosaminoglycan chains allowing them to act as peptide receptors or co-receptors [4] , [5] , [6] . As syndecan-3 has been shown to act as an alternative receptor for GDNF [6] , a peptide that can both increase and reduce drug-seeking behavior [14] , and as GDNF is expressed in the LH [15] , we investigated whether the effects of syndecan-3 in regulating cocaine intake were mediated by GDNF. As GDNF has been shown to attenuate acquisition of cocaine self-administration in rats [16] , we injected cocaine-self-administering mice with a GDNF-expressing AAV after acquisition of cocaine self-administration ( Fig. 5a ). To this end, we used a double-stranded AAV vector that is more rapidly expressed than conventional single stranded AAV. We observed that AAV-GDNF significantly and dramatically increased cocaine intake in syndecan-3 KO mice at the training dose, although it did so only marginally in WT mice ( Fig. 5b ). AAV-GDNF shifted upwardly the dose-response curve significantly both in syndecan-3 KO and WT mice, but considerably more in syndecan-3 KO mice than in wild-type mice ( Fig. 5c ). This suggested that LH syndecan-3 limits compulsive cocaine intake by countering the action of GDNF through its canonical receptor complex comprising the high-affinity binding receptor GFR-α1 and the signaling transmembrane receptor tyrosine kinase c-Ret. Consistent with this interpretation, we observed that administration of the c-Ret inhibitor vandetanib [17] selectively abolished the increased cocaine self-administration induced by AAV-GDNF in syndecan-3 KO mice ( Fig. 5d ). Thus, LH syndecan-3 acts as an addiction-resilience factor by modulating the effects of GDNF on cocaine seeking. 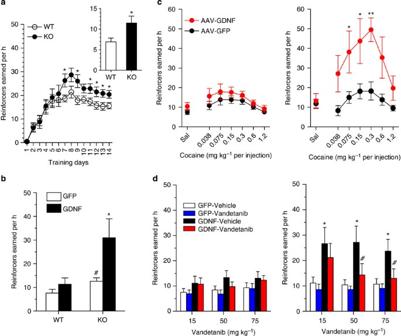Figure 5: LH syndecan-3 modulates the effect of GDNF on cocaine intake. (a) Acquisition of cocaine self-administration before intra-LH infusion of AAV-GDNF: syndecan-3 KO mice showed a higher level of cocaine intake at the training dose (FR1) than wild-type mice (WT). RM two-way ANOVA: Test sessionF(13,442)=25.39,P<0.0001; GenotypeF(1,442)=4.481,P=0.0417. *P<0.05 compared with wild-type mice (n=18 for each genotype). Inset: syndecan-3 KO mice also showed higher lever pressing rates than wild-type mice after switching to FR5 schedule (t=2.36,P=0.021 byt-test). (b) Intra-LH infusion of an AAV vector expressing GDNF (AAV-GDNF) increased cocaine self-administration at the training dose (FR5). Two-way ANOVA showed a significant main effects of AAV-GDNF (F(1,23)=7.206,P=0.013) and genotype (F(1,23)=8.881,P=0.007). *P<0.05 AAV-GFP versus AAV-GDNF of KO mice;#P<0.05 syndecan-3 KO vs wild type mice infused with AAV-GFP (by LSD post hoc test). (c) Intra-LH infusion of AAV-GDNF upward-shifted the dose-response curve (FR5) in wild-type mice (left panel) and syndecan-3 KO mice (right panel). Left panel: DoseF(6,112)=3.573,P=0.003; AAV-GDNFF(1,112)=5.959,P=0.016. Right panel: DoseF(6,77)=3.585,P=0.004; AAV-GDNFF(1,77)=33.01,P<0.0001. *P<0.05 and **P<0.01 AAV-GFP versus AAV-GDNF (n=6–9, by LSD post-hoc test). (d) The c-Ret inhibitor vandetanib (15, 50 and 75 mg kg−1, s.c.) did not modify cocaine intake in wild-type mice infused with either AAV-GFP or AAV-GDNF in the LH (left panel), but selectively reduced cocaine self-administration in syndecan-3 KO mice infused with AAV-GDNF (right panel). Left panel: in wild-type mice, RM two-way ANOVA did not reveal significant main vandetanib effect at any dose of 15 mg kg−1(F(1,13)=0.165;NS), 50 mg kg−1(F(1,13)=3.435;NS) and 75 mg kg−1(F(1,13)=0.095; NS). Right panel: in syndecan-3 KO mice, RM two-way ANOVA showed a significant main effect of vandetanib at 15 mg kg−1(F(1,11)=5.979;P=0.033), 50 mg kg−1(F(1,11)=9.694;P<0.01 with significant interactionF(1,11)=5.412;P=0.04), and 75 mg kg−1(F(1,11)=24.08;P<0.001 with significant interactionF(1,11)=12.65;P=0.005). *P<0.05 AAV-GFP versus AAV-GDNF;#P<0.05 vehicle versus vandetanib group (n=6–7, by LSDpost-hoctest). All data are presented as mean±s.e.m. Figure 5: LH syndecan-3 modulates the effect of GDNF on cocaine intake. ( a ) Acquisition of cocaine self-administration before intra-LH infusion of AAV-GDNF: syndecan-3 KO mice showed a higher level of cocaine intake at the training dose (FR1) than wild-type mice (WT). RM two-way ANOVA: Test session F (13,442) =25.39, P <0.0001; Genotype F (1,442) =4.481, P =0.0417. * P <0.05 compared with wild-type mice ( n =18 for each genotype). Inset: syndecan-3 KO mice also showed higher lever pressing rates than wild-type mice after switching to FR5 schedule ( t =2.36, P =0.021 by t -test). ( b ) Intra-LH infusion of an AAV vector expressing GDNF (AAV-GDNF) increased cocaine self-administration at the training dose (FR5). Two-way ANOVA showed a significant main effects of AAV-GDNF ( F (1,23) =7.206, P =0.013) and genotype ( F (1,23) =8.881, P =0.007). * P <0.05 AAV-GFP versus AAV-GDNF of KO mice; # P <0.05 syndecan-3 KO vs wild type mice infused with AAV-GFP (by LSD post hoc test). ( c ) Intra-LH infusion of AAV-GDNF upward-shifted the dose-response curve (FR5) in wild-type mice (left panel) and syndecan-3 KO mice (right panel). Left panel: Dose F (6,112) =3.573, P =0.003; AAV-GDNF F (1,112) =5.959, P =0.016. Right panel: Dose F (6,77) =3.585, P =0.004; AAV-GDNF F (1,77) =33.01, P <0.0001. * P <0.05 and ** P <0.01 AAV-GFP versus AAV-GDNF ( n =6–9, by LSD post-hoc test). ( d ) The c-Ret inhibitor vandetanib (15, 50 and 75 mg kg −1 , s.c.) did not modify cocaine intake in wild-type mice infused with either AAV-GFP or AAV-GDNF in the LH (left panel), but selectively reduced cocaine self-administration in syndecan-3 KO mice infused with AAV-GDNF (right panel). Left panel: in wild-type mice, RM two-way ANOVA did not reveal significant main vandetanib effect at any dose of 15 mg kg −1 (F (1,13) =0.165; NS ), 50 mg kg −1 (F (1,13) =3.435; NS ) and 75 mg kg −1 (F (1,13) =0.095; NS). Right panel: in syndecan-3 KO mice, RM two-way ANOVA showed a significant main effect of vandetanib at 15 mg kg −1 (F (1,11) =5.979; P =0.033), 50 mg kg −1 ( F (1,11) =9.694; P <0.01 with significant interaction F (1,11) =5.412; P =0.04), and 75 mg kg −1 ( F (1,11) =24.08; P <0.001 with significant interaction F (1,11) =12.65; P =0.005). * P <0.05 AAV-GFP versus AAV-GDNF; # P <0.05 vehicle versus vandetanib group ( n =6–7, by LSD post-hoc test). All data are presented as mean±s.e.m. Full size image Syndecans are type I transmembrane proteins found at the cell surface of adherent cells that are increasingly recognized as modulating ligand–receptor interactions at the cell surface in addition to functioning as structural components of the extracellular matrix. Our results show that syndecan-3 signaling in the LH has an inhibitory role on motivation to self-administer cocaine. While syndecan-3 is a co-receptor for certain ligands and enhances the formation of their receptor-signaling complexes [4] , our findings demonstrate another role of syndecan-3 as an alternative GDNF receptor that counterbalances the effects of GDNF on its high-affinity receptor complex, GFR-α1/c-Ret. The syndecan-3 ligand pleiotrophin has been recently shown to exert differential actions on prostate cells acting through syndecan-3 or its conventional receptor RPTβ/ζ [7] . Thus, syndecan-3 may have a general role counterbalancing the effects of some of its ligands on their conventional receptors. This new mechanistic concept suggests that modulating the relative actions of specific syndecan-3 ligands on syndecan-3 versus their conventional receptors can be a novel therapeutic approach in multiple settings beyond cocaine addiction. The identification of molecular determinants of resilience to addiction is a novel conceptual approach to the search for effective therapeutic targets for treating addiction [18] , [19] . The results of the present study provide the rationale for therapeutic strategies aimed at strengthening syndecan-3 signaling for the treatment of cocaine abuse. In particular, we observed that LH syndecan-3 regulates cocaine-reinforcing properties, but syndecan-3 null and wild-type mice did not differ in their responses to passively administered cocaine such as locomotor activation and the cardiovascular effects of cocaine. The effect of syndecan-3 on motivation for cocaine was specific as syndecan-3 null and wild-type mice did not differ in preference for a natural reward like sucrose. Thus, syndecan-3 in the LH may be targeted to control motivation for cocaine without impairing their motivation toward natural reinforcers. These results also highlight a key role for the LH in cocaine reward and motivation. Classic studies have implicated the LH in reward and motivation [20] , [21] . The LH is interconnected to key reward-related regions such as the NAc, central and medial amygdala, the bed nucleus of the stria terminalis and the medial prefrontal cortex [22] , [23] , [24] . Thus, it is well positioned to integrate sensory and interoceptive stimuli and mediate motivated behaviors such as drug seeking [25] , [26] . Electrical intracranial self-stimulation (ICSS) in the LH is highly reinforcing and is potentiated acutely by cocaine and other drugs of abuse, and decreased during withdrawal [27] . A key role of LH neurons in motivation is supported by manipulations that do not affect fibers of passage [28] , [29] , [30] , as well as by gene expression evidence of cocaine-induced remodeling of LH circuitry [9] . The present results support the notion that neural circuits involving the LH contribute to drug reward and indicate that syndecan-3 exerts a key activity in these circuits. The present data provide a novel neurobiological mechanism by which the LH regulates cocaine reward and suggest that syndecan-3-dependent signaling in the LH is a novel addiction-resilience mechanism. Identification of factors contributing to resistance to addiction may be of equal or even greater importance as identification of addiction-vulnerability factors in the hunt for means of returning an organism to hedonic homeostasis, and in seeking future targets for novel treatments. Lastly, we also identify a molecular mechanism for syndecan-3 as a modulator of effects of GDNF, which may be exploited therapeutically for the treatment of cocaine abuse. Intravenous cocaine self-administration in the rat The use of animals was approved by the TSRI Institutional Animal Care and Use Committee (IACUC) with Protocol Number 08-0017 and 08-0017-2. Intravenous cocaine self-administration was conducted as described earlier [9] . Briefly, male Wistar rats (280–340 g) were prepared with a chronic i.v. jugular catheter and trained for 7 days to press a lever to obtain food pellets. After 2 days of food training, rats were tested for cocaine self-administration at FR1 with 1-h access (250 μg per injection in a volume of 0.1 ml delivered in 4 sec) and then assigned to two balanced groups. One group was switched to 6-h access to self-administration per day (LgA rats), while the other was kept at 1-h access (ShA group). For intravenous cocaine self-administration in the rhesus monkeys ( Macaca mulatta , macaque), animals were surgically prepared and trained to self-administer cocaine at a unit dose of 0.1 mg kg −1 per injection (FR1). Mouse jugular vein catheterization Male syndecan-3 KO mice in a C57BL/6J [12] were housed in a climate-controlled vivarium on a 12 h reversed light–dark cycle (lights on 9:00), and food and water were provided ad libitum through the study. Mice were implanted with intravenous jugular catheters under anesthesia with ketamine (Ketaset, 80 mg kg, i.p., Fort Dodge Animal Health) and xylazine (16 mg/kg, i.p., Butler Animal Health). Catheters were made from a 6 cm length of silastic tubing fitted to a port consisting of a flanged cannula with a plastic disk (Plastics One). The catheter port was covered with silicon adhesive sealant. During the surgery, the catheter tubing was threaded subcutaneously, with the external port exiting the midscapular region and a 1-cm length of the tip was inserted into the right external jugular vein. The catheter was tied into the vein proximally with silk suture and filled with a 25-μl heparinized saline solution (30 USP U ml −1 , APP pharmaceuticals, LLC) containing cefazolin (100 mg ml −1 , Apotex Corp.). The catheters were flushed daily with the same solution for 3 additional days and thereafter with the heparinized saline solution without antibiotic. The mice were allowed to recover from the surgery for at least a week. Intravenous cocaine self-administration in the mouse Mice were trained to press a lever in an operant chamber (Med Associates) for intravenous injections of cocaine (0.6 mg kg −1 per injection) under a FR1 time-out 20-s schedule (FR1TO20) during 1 h daily sessions, 5 days per week. The concentration of cocaine was 1.2 mg ml −1 and the injection volumes were adjusted for each mouse’s body weight (0.5 ml kg −1 ) by adjusting the infusion durations. Criterion for acquisition of cocaine self-administration was a stable level of cocaine self-administration behavior (a minimum of 10 reinforcers earned per session with at least 70% of total responses on the active lever) over two consecutive sessions (±20%). After attainment of acquisition, a full dose–effect study was then performed on a FR5 or a PR schedule [31] . In the FR5 study, the response requirement was gradually increased to FR5 at the training dose (0.6 mg kg −1 per injection), and once a stabilized self-administration behavior was reached, each of the unit doses (1.2, 0.6, 0.3, 0.15, 0.075 and 0.038 mg kg −1 per injection) was tested in descending order in 1-h daily sessions with two sessions for each dose. The same unit dose–effect analysis of the reinforcing efficacy of cocaine was performed using the PR schedule. The PR formula was: 5 × exp(reinforcer number × 0.2)−5, which yields values of 1, 2, 4, 6, 9, 12, 15, 20, 25, 32, 62, 77, 95, 118, 145, et cetera . The breakpoint was defined as the step value associated with the last completed ratio after a 20 min limited hold. Under both the FR5 and PR schedules, each dose was tested during 1-h daily sessions for two test sessions. The numbers of reinforcers earned, total cocaine intake and breakpoints from the mean of two consecutive sessions at each dose were analyzed by repeated measure (RM) of two-way ANOVA. At the end of experiment, catheter patency was verified with solution of ketamine and midazolam (0.25 mg and 0.0125, mg in 50 μl), and mice with a defective catheter were excluded from statistical analysis. Drug The c-Ret kinase inhibitor Vandetanib was purchased from the LC Laboratories (Woburn, MA) and dissolved in DMSO/PEG200/Saline (for 15 mg kg −1 , the ratio was 1:5:4; for 50 and 75 mg kg −1 , the ratio was 3.3:5:1.7). The vehicle and Vandetanib solutions were injected (5 ml kg −1 , s.c.) 1 h prior to the self-administration tests. Sucrose intake test Sucrose consumption was examined by a two-bottle choice procedure [32] . Mice (11 KO and 12 WT mice) were given 1 week to acclimate to individual housing conditions and drinking from two sipper tubes. During this period, they were assessed for baseline water consumption in 24-h daily drinking sessions. Mice were then given a choice between one bottle with sucrose and one bottle of water. The sucrose concentration was increased from 0.001% to 20% (0.001, 0.01, 0.1, 1, 2.5, 5, 10 and 20%) with 2 days access at each concentration. The position of the two bottles was switched every day to control potential side preferences. Mice were weighted daily and sucrose and water intakes (g kg −1 ) were measured every 24 h, 7 days per week. Locomotor activity and heart rate measurements Locomotor activity was measured in open field activity chamber (43 × 21.5 × 30 cm, Med Associates). During baseline session, all mice were injected saline (i.p.) and individually tested for 15 min. In acute cocaine session, mice were injected cocaine (6, 12 or 18 mg kg −1 , i.p.). Ambulatory distance from the last three of six baseline sessions were averaged to determine basal activity level and compared with acute cocaine session. Heart rate was determined electrophysiologically by electrocardiogram (EKG) by subcutaneous insertion of two electrodes behind the left foreleg and the other in front of the right hindleg. Recordings were made through an Axon 2000B amplifier. Microinfusion of AAV AAV vectors (AAV2 serotype) expressing either a bicistronic transcript including the open reading frames of syndecan-3 and GFP linked through a IREs (AAV-Snd3) or expressing GFP alone (AAV-GFP) from a CMV promoter were prepared according to conventional protocols. A shedding-resistant allele was used for AAV-Snd3 in which 30 AA of the juxtamembrane segment were replaced with the corresponding sequence of syndecan-1, which is not cleaved in the brain and acts as a constitutively active syndecan-3 (ref. 33 ). As GDNF attenuates acquisition of cocaine self-administration in rats [16] , we used a previously reported double-stranded AAV vector to deliver GDNF [34] , as it express more rapidly than conventional single stranded AAV vectors and, therefore, it could be administered after acquisition if cocaine self-administration. Animals were anesthetized as described earlier for intra-LH virus injections. Briefly, mice were immobilized in a stereotaxic frame in the flat-skull position (Kopf Instruments) and a bilateral stainless steel injector (33 ga, extended 1 cm below the tip of a 26-ga sleeve tubing) was lowered into the LH (coordinates: −0.94 mm anterior to bregma, ±1.2 mm lateral and −5.4 mm ventral to skull surface at bregma). The AAV solution (10 genomic particles per ml [13] ) was delivered slowly through the injector by a syringe pump (0.5 μl each at a flow rate of 0.05 μl per min, Kd Scientific). The injector remained in the place for at least 10 min and then was withdrawn slowly to avoid backflow of the virus. AAV expression could be detected for >1 year after infusion, as shown in Fig. 1e . For detection of GFP expression, 40-μm cryostat sections were immunoreacted with an anti-GFP antibody (CloneTech; Catalog number: 632381) at a dilution of 1:500 overnight, followed by incubation with an FITC-labeled secondary antibody for 1 h. Microarray analyses Total LH RNA from rat self-administering cocaine and cocaine-naive controls were analyzed using RNU34 Affymetrix GeneChip arrays. Expression measurements were normalized using gcrma in R-2.11.1 and the values were adjusted for the heatmap by subtracting their means across all samples and divided by their s.d., z =( x −mean)/std. We also filtered out probe sets that were not called ‘present’ in at least one condition by MAS5 detection, using mas5calls in R-2.11.1 ( Supplementary Data 1 ). Gene set enrichment analysis GSEA [35] was used to test the enrichment of genes involved in syndecan’s signaling in a gene signature of response to cocaine self-administration in rats (NCBI GEO accession no. GSE3016 ). GSEA was run using 30 genes suggested by literature as being involved in syndecan’s signaling ( Supplementary Table S1 ). These genes were tested against a ranked list of expressed genes in the gene expression profiles sorted by the absolute value of their differential expression ( t -statistic) between cocaine-exposed and control samples in the LH. Significance testing was performed by shuffling the gene-labels 1,000 times. Western blots Dissected hypothalamic tissues were homogenized in 300 μL of ice-cold heparitinase buffer (50 mM Hepes pH6.5, 50 mM NaOAc, 150 mM NaCl, 5 mM CaCl 2 ) containing the complete protease inhibitor cocktail (PIC, Roche) with a Polytron. The homogenates were centrifuged at 1,4000, r.p.m. for 45 min at 4 °C. The heparitinase buffer-soluble material was removed, and the resulting pellets were resuspended with 1% Triton X-100 in heparitinase buffer+PIC, incubated on ice for an hour and centrifuged as above. The Triton X-extracted fraction was then treated with heparitinase+chondroitinase ABC lyase (Sigma) for a total of 4 h at 37 °C, and the digestion was stopped with the SDS-PAGE 6 × sample buffer. Aliquots of the digested protein extracts were then subjected to SDS gel electrophoresis and electrophoretically transferred to Immobilon P membrane (Millipore). Blots were incubated with anti-syndecan antibody targeting the syndecan ectodomain. Statistical analysis All behavioral data were analyzed by two-way ANOVA with repeated measures on dose or test session, followed by least significant difference (LSD) tests (SPSS software 11.0). How to cite this article: Chen, J. et al. Hypothalamic proteoglycan syndecan-3 is a novel cocaine addiction resilience factor. Nat. Commun. 4:1955 doi: 10.1038/ncomms2955 (2013).